Non-canonical function of spindle assembly checkpoint proteins after APC activation reduces aneuploidy in mouse oocytes The spindle assembly checkpoint (SAC) prevents aneuploidy by coupling anaphase onset, through anaphase-promoting complex (APC) activation, with chromosome attachment to spindle microtubules. Here, we examine APC activity in oocytes, noted for their susceptibility to chromosome mis-segregation during the first meiotic division (MI). We find that MI oocytes only contain sub-maximal APC activity, measured through cyclin B1–GFP degradation, because inhibition of SAC proteins when the APC is normally fully active increases cyclin B1 degradation twofold and reduces the length of this division by 2 h. In addition, inhibiting the SAC component Mps1 only when the APC is already active increases aneuploidy rates in the resulting egg by up to 30%. We therefore establish that the activities of SAC proteins and the APC co-exist in oocytes, and such concurrence has a vital role in reducing aneuploidy rates by extending MI, probably by allowing time for numerous erroneous microtubule attachments to be corrected. In the divisions associated with both mitosis and meiosis, the timing of chromosome segregation is regulated by the spindle assembly checkpoint (SAC) in order to prevent the creation of aneuploid daughter cells or embryos [1] , [2] . This ubiquitous checkpoint pathway does this by coupling the proper attachment of kinetochores to spindle microtubules with anaphase onset. In prometaphase, the SAC is active: a state in which a diffusible anaphase-promoting complex (APC) inhibitor is generated from free kinetochores that act as a platform on which the most upstream SAC components, such as Mps1, are assembled [1] , [3] . In the ‘template model’ of SAC activation, a molecular rearrangement of Mad2 occurs when it is recruited to the kinetochore [4] , [5] , a process needed to generate a diffusible and potent APC inhibitor, the mitotic checkpoint complex (MCC), and thus prevent the degradation of APC substrates critical for M-phase exit such as cyclin B1 and securin [6] . SAC activity declines as kinetochores attach to spindle microtubules—a process likely involving disassembly and removal of the SAC components from attached kinetochores [7] . In mitosis, recent work has demonstrated that APC inhibition by the SAC can be graded, and correlates with the remaining amount of kinetochore bound Mad2 (refs 8 , 9 ). As in all mammals, oocytes of mice show a particularly protracted MI, in which bivalents—recombined homologous chromosome pairs—are segregated over a period lasting many hours. Despite these differences to mitosis, the division remains APC dependent and has a full complement of SAC proteins, whose loss brings forward the timing of APC activity and significantly raises aneuploidy rates [10] , [11] , [12] , [13] , [14] , [15] , [16] . A robust checkpoint should not permit APC-mediated cyclin B1 or securin degradation until all chromosomes achieve bipolar microtubule attachment (biorientation). However, misaligned bivalents that have incorrect microtubule attachment and so are not biorientated, exist simultaneously with an active APC and meiotic progression [17] , [18] , [19] , [20] . This lack of correlation between onset of APC activation and biorientation prompted us to examine the control that the SAC had on APC activity throughout MI. Here we find that such lack of correlation, which would potentially act to drive up rates of chromosome mis-segregation, is mitigated by a delay to anaphase brought about by SAC proteins inhibiting full APC activation during meiotic exit. This reduction makes MI longer by 2 h, and significantly increases aneuploidy if bypassed. MI progression is uncoupled from bivalent biorientation To examine how the SAC behaves in oocytes, germinal vesicle (GV) stage mouse oocytes, equivalent to G2, were microinjected with cRNA encoding Histone2B-mCherry to label chromatin, and CenpC-GFP for kinetochores. Three-dimensional confocal imaging of live cells was used to examine the position of bivalents relative to the spindle equator following nuclear envelope breakdown (NEB; Fig. 1a ). Biorientation of chromosomes was inferred by (a) the position of the bivalent at the spindle equator that must be maintained by balanced attachment to each spindle pole, and (b), the distance apart of the two sister kinetochore pairs, referred to here as ‘bivalent stretch’, which would increase in proportion to the pulling forces exerted by kinetochore-bound microtubules from opposing poles. Misaligned bivalents, which are not initially near the spindle equator, are a common feature of oocytes at ~6 h after nuclear envelope breakdown (NEB) [17] , but almost all achieve biorientation before anaphase onset ( n =11/12), judged by their movement to the equator and the increased level of stretch that is observed between sister kinetochore pairs ( Fig. 1b ; grey-marked bivalent at 06:25 h; Supplementary Fig. 1 ; Supplementary Movie 1 ). However, some bivalents, even within the same oocyte, can remain misaligned during MI ( Fig. 1b ; blue-marked bivalent; Supplementary Fig. 1 ; Supplementary Movie 1 ), and fail to develop lasting stretch between the sister kinetochore pairs. These non-aligned bivalents, which lack biorientation, do not block anaphase, but instead mis-segregate at MI completion. 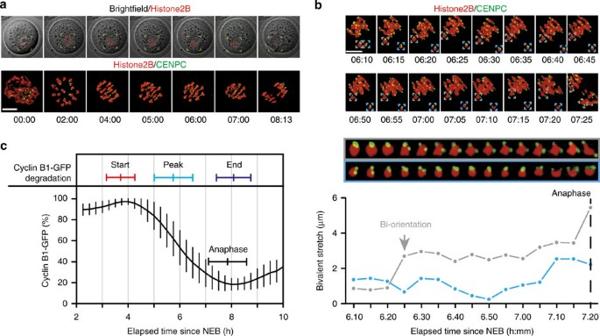Figure 1: Bivalents that fail to biorientate do not block MI and can undergo nondisjunction. (a) Meiotic progression in an oocyte from NEB to anaphase onset. Upper row, oocyte with bivalents labelled with histone 2B-mCherry; yellow square, region imaged in more detail (lower row) by chromosome tracking. (b) Oocyte imaged with two non-biorientated bivalents (grey, blue boxes; enlarged below) in a 75-min period before anaphase. Maximal bivalent stretch, measured as the distance apart from the sister kinetochores pairs and regarded as a measure of biorientation, is achieved in one of these non-aligned bivalents (grey) but not in the other (blue). (c) Cyclin B1-GFP levels (mean and s.d.n=48 oocytes), normalized with respect to maximal levels, during exit from MI. From this plot were calculated the time of cyclin B1 degradation onset (red; mean and s.d.), its maximal rate (blue) and the timing of its completion (purple). Oocytes expressed cyclin B1–GFP and histone 2B-Cherry, from which the time timing of anaphase was measured (black). (a,b) Scale bars, 10 μm, times are hh:mm. Figure 1: Bivalents that fail to biorientate do not block MI and can undergo nondisjunction. ( a ) Meiotic progression in an oocyte from NEB to anaphase onset. Upper row, oocyte with bivalents labelled with histone 2B-mCherry; yellow square, region imaged in more detail (lower row) by chromosome tracking. ( b ) Oocyte imaged with two non-biorientated bivalents (grey, blue boxes; enlarged below) in a 75-min period before anaphase. Maximal bivalent stretch, measured as the distance apart from the sister kinetochores pairs and regarded as a measure of biorientation, is achieved in one of these non-aligned bivalents (grey) but not in the other (blue). ( c ) Cyclin B1-GFP levels (mean and s.d. n =48 oocytes), normalized with respect to maximal levels, during exit from MI. From this plot were calculated the time of cyclin B1 degradation onset (red; mean and s.d. ), its maximal rate (blue) and the timing of its completion (purple). Oocytes expressed cyclin B1–GFP and histone 2B-Cherry, from which the time timing of anaphase was measured (black). ( a , b ) Scale bars, 10 μm, times are hh:mm. Full size image To study the activity of the APC during the period of bivalent non-alignment, whole-cell fluorescence levels were imaged in oocytes injected with cyclin B1–GFP and histone2B-mCherry cRNA. Following NEB, an initial period of cyclin B1 synthesis was measured, such that maximal fluorescence was reached at 3.7±0.5 h (mean±s.d. ; n =48 oocytes; all timings were measured as elapsed time since NEB; Fig. 1c ). This maximal fluorescence was normalized to 100%, to allow comparison between oocytes. For each experiment only oocytes with an absolute maximum fluorescence within a narrow range were analysed, to ensure that exogenous cyclin B1 levels were similar between cells ( Supplementary Fig. 2 ). There followed on average a 4.5-h period of cyclin B1 degradation, which was complete by 8.2±0.7 h ( n =48); anaphase onset occurred 0.4 h before the minimum level ( Fig. 1c ). The maximum rate of cyclin B1 loss, 32.3±5.0% h −1 ( n =48), was achieved at about 6 h after NEB (5.7±0.7 h), which was taken in all subsequent experiments as the time of maximal APC activity. It concerned us that exit from MI appeared to be initiated through APC activation, at a time when some bivalents were clearly not biorientated. This may be explained by cyclin B1 degradation occurring through a pathway independent of SAC–APC control. In such a situation, the APC is still held in check by the SAC, but an APC-independent pathway is responsible for cyclin B1 degradation. However, this seems unlikely, given cyclin B1 degradation is dependent on the presence of its D-box degron [6] , and is blocked by loss of the APC activator Cdc20 (refs 21 , 22 )—factors that strongly support APC-mediated degradation. Moreover, cyclin B1 degradation is blocked in a Mad2-dependent manner by addition of spindle poisons [23] and oocytes arrest in MI following Mad2 overexpression [11] , [24] —factors that support the involvement of the SAC. To explain why the APC is active towards cyclin B1 in the presence of non-aligned chromosomes, we considered how SAC activity might be regulated during meiotic exit. Previously, we observed that during the time of APC activity, Mad2 was still retained on the kinetochores of both aligned and non-aligned bivalents [17] . This level was significantly lower than that present in the early prometaphase when cyclin B1 is stable. In addition, we had shown that despite recruiting more Mad2, non-aligned bivalents did not significantly delay anaphase onset. This suggests that small numbers of non-aligned bivalents do not produce a SAC signal sufficient to inhibit the APC and so stabilize cyclin B1. The continued presence of low levels of kinetochore-associated Mad2 on bivalents, independent of their biorientation, prompted us to investigate if SAC proteins were still making some contribution to APC inhibition and influencing the duration of MI exit. CDK1 inhibition increases cyclin B1 degradation rate To determine the factors influencing MI exit, we re-examined the shortening of MI caused by the CDK inhibitor roscovitine [17] . Its addition to oocytes at 6 h after NEB shortened MI by 1.1 h (±0.1 h, n =36), as measured by polar body extrusion. This acceleration was previously suggested to be due to a rapid dephosphorylation of CDK1 substrates by phosphatases such as PP2A [25] . This seemed plausible because anaphase is dependent on low CDK1 activity [26] . However, anaphase is also dependent on other factors such 26S proteasomal activity, needed to degrade APC ubiquitin-tagged substrates and resolution of cohesin, a process that requires activation of the protease separase through APC-mediated destruction of its inhibitory chaperone securin. Rapid exit from MI could therefore have been due to either increased APC or proteasome activity. To examine this further, using oocytes expressing cyclin B1–GFP, it was tested if cyclin B1 degradation could be increased following CDK1 inhibition, and here the more potent CDK inhibitor flavopiridol was used in preference to roscovitine ( Supplementary Fig. 3 ). Drug addition was at 6 h after NEB, a time point associated with maximal cyclin B1 degradation ( Fig. 1c ). At this time, the rate of degradation is linear, which allows comparison of degradation rates before and after drug addition. In addition, this time is also associated with a low level of cyclin B1–GFP synthesis ( Supplementary Fig. 4a,b ), such that any observed change in cyclin B1–GFP fluorescence can be attributed almost entirely to the much greater rate of APC-mediated degradation (~2% h −1 synthesis, n =32 versus ~30% h −1 degradation, n =31). Interestingly, flavopiridol addition caused cyclin B1 degradation rates to increase twofold—from 28±8% h −1 to 55±10% h −1 ( n =37; P <0.001, Tukey’s Multiple Comparison Test; Fig. 2a ), but no such increase was observed with a vehicle control. The acceleration in timing of polar body extrusion following roscovitine/flavopiridol addition is therefore accounted for not only by CDK inhibition but also by an increase in the activity of the APC, or indeed the 26S proteasome. 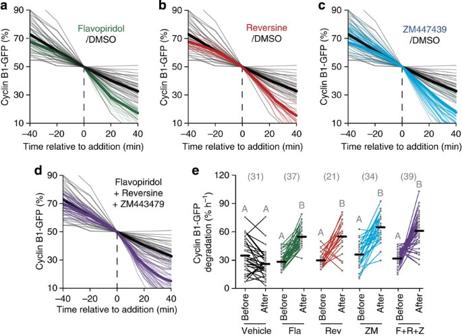Figure 2: Doubling of cyclin B1 degradation rates in oocytes by chemical inhibitors of the SAC. (a–d) Normalized cyclin B1–GFP intensity plotted against time relative to chemical addition (minutes). Vehicle controls (DMSO) are indicated in black; flavopiridol, green; reversine, red; ZM447439, blue; all chemical inhibitors together, purple. Bold lines are means; individual traces indicated by pale lines. (e) Cyclin B1-GFP degradation rates in oocytes immediately before and after chemical additions (a–d). Black horizontal lines are means; coloured lines connect data points from the same oocyte; numbers of oocytes are indicated in parenthesis; different letters indicate significant difference between groups (P<0.001; analysis of variance). Figure 2: Doubling of cyclin B1 degradation rates in oocytes by chemical inhibitors of the SAC. ( a – d ) Normalized cyclin B1–GFP intensity plotted against time relative to chemical addition (minutes). Vehicle controls (DMSO) are indicated in black; flavopiridol, green; reversine, red; ZM447439, blue; all chemical inhibitors together, purple. Bold lines are means; individual traces indicated by pale lines. ( e ) Cyclin B1-GFP degradation rates in oocytes immediately before and after chemical additions ( a – d ). Black horizontal lines are means; coloured lines connect data points from the same oocyte; numbers of oocytes are indicated in parenthesis; different letters indicate significant difference between groups ( P <0.001; analysis of variance). Full size image The above experiment suggested that during the normal course of MI, APC-mediated cyclin B1 degradation is not maximal. Identifying the mechanism for this is difficult because CDK1 has a number of substrates and its inhibition potentially affects many cellular pathways. However, we do know that the increase is not dependent on the APC co-activator Fzr1/Cdh1, which is present in oocytes [27] , [28] because Fzr1 knockout oocytes showed a similar increase in cyclin B1 degradation when treated with flavopiridol ( Supplementary Fig. 5 ). Mps1 or Aurora kinase inhibition raises APC activity Mps1 kinase is an essential component of the SAC because of its ability to bind free kinetochores and recruit SAC components to the kinetochore [29] and to inhibit the APC by MCC generation [30] . In addition, it is a CDK1 substrate, and requires this kinase for its own activity [31] . Therefore, one attractive hypothesis is that during MI exit CDK1 reduces APC activity through Mps1, but not at a level sufficient to prevent anaphase. In order to test if Mps1 activity contributes continuously in MI exit to decrease APC activity, reversine, an Mps1 kinase inhibitor [32] , was used ( Supplementary Fig. 3 ). As with flavopiridol, an approximate twofold increase in APC activity was measured following reversine addition at 6 h after NEB in oocytes expressing cyclin B1, when the APC is otherwise maximally active (before reversine: 30±9% h −1 ; after reversine: 55±17% h −1 ; n =21; P <0.001, Tukey’s multiple comparison test; Fig. 2b ). The above findings suggest that APC activity is sub-maximal during MI exit, due to the negative influence of Mps1 kinase. To explore if other SAC components were involved, a third chemical intervention was made using ZM447439, a pan-aurora kinase inhibitor ( Supplementary Fig. 3 ). In most cells Aurora B is thought to localize to the inner centromere, where it destabilizes low-tension, incorrect microtubule attachments [33] , [34] . In oocytes, this function is likely achieved by the meiotic specific isoform Aurora C [35] . The role of Aurora kinase in the SAC response itself, being distinct from its role helping establish correct biorientation, has been demonstrated previously in somatic cells [36] , [37] . In addition, confirming Aurora kinase’s meiotic role in SAC signalling, ZM447439 in mouse oocytes can be used to overcome a SAC-imposed arrest induced by the spindle poison nocodazole [12] . When added to oocytes at 6 h after NEB, the time when APC activity is normally maximal with respect to degrading cyclin B1, ZM447439 increased the rate of loss of this APC substrate from 36±12% h −1 to 65±13% h −1 ( n =34; P <0.001, Tukey’s multiple comparison test; Fig. 2c )—approximately the same increase as that with flavopiridol or reversine. The observation that flavopiridol, reversine or ZM447439 addition all raised cyclin B1 degradation rates by similar amounts suggested that they may work on the same pathway, and here we are proposing this is alleviation of partial APC inhibition by SAC proteins imposed during MI exit. Therefore, we wanted to examine if there would be any synergistic effect of the three chemicals added together, a finding that would counter this hypothesis. The combined effect on APC activity of simultaneous addition of the three chemicals was measured and found to have no additive or synergistic effect ( Fig. 2d ). Instead, cyclin B1 had the same degradation rate as that achieved by individual chemical addition, increasing from 32±9% h −1 to 61±19% h −1 ( n =39). This increase was not significantly different from any of the three inhibitors used separately ( Fig. 2e ). Mad2 antibody increases cyclin B1 degradation rate One drawback of the approach used so far, in trying to examine APC activity at a time when it is maximal 6 h after NEB, is that it relied on chemical intervention. Therefore, to inhibit the SAC non-pharmacologically a functionally inhibitory antibody against Mad2 (ref. 38) [38] was used. Despite our extensive experience of performing microinjections at other meiotic timepoints (<5% cell death), we consistently found antibody microinjection at this time challenging because it was associated with extensive levels of cell lysis (>85% cell death). In those surviving oocytes ( n =16/110), a heat-treated control antibody injection significantly reduced cyclin B1–GFP degradation rates ( n =7; P =0.0485, paired t -test; Fig. 3a,b ). A drop was to be expected given the sensitivity of this time point to microinjection and the likely resulting disruption of cell processes. In contrast, however, microinjection of the native antibody significantly increased APC activity from 29% h −1 to 46% h −1 ( n =9; P =0.0015, paired t -test; Fig. 3a,b ). 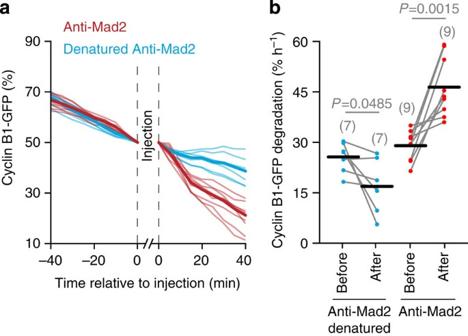Figure 3: Mad2 inhibition raises cyclin B1 degradation rates in oocytes. (a) Cyclin B1–GFP levels in oocytes during exit from MI at 6 h after NEB before and after injection of either Mad2 (red) or heat-denatured Mad2 (blue) antibody. Fluorescence was normalized to the time of injection (set to 50%). Microinjections were performed over 10–15 min. (b) Cyclin B1–GFP degradation rates in a 20-min period immediately before and after microinjections. Numbers of oocytes injected are in parenthesis; points linked by grey lines indicate same oocytes;P-values are pairedt-tests. Figure 3: Mad2 inhibition raises cyclin B1 degradation rates in oocytes. ( a ) Cyclin B1–GFP levels in oocytes during exit from MI at 6 h after NEB before and after injection of either Mad2 (red) or heat-denatured Mad2 (blue) antibody. Fluorescence was normalized to the time of injection (set to 50%). Microinjections were performed over 10–15 min. ( b ) Cyclin B1–GFP degradation rates in a 20-min period immediately before and after microinjections. Numbers of oocytes injected are in parenthesis; points linked by grey lines indicate same oocytes; P- values are paired t -tests. Full size image Taken together, all the above data show that the APC is not maximally active in MI, at the time when maximal cyclin B1 degradation is normally measured. This appears due to persistent activity of SAC proteins, which effectively halves the rate of APC substrate degradation. At this point, we can also rule out the possibility that the observations are based on increased 26S proteasomal activity, rather than the APC, because the SAC proteins Mad2, Aurora kinase and Mps1 are only known to influence the latter. APC inhibition by SAC proteins requires bivalents The source of the APC inhibition, based on the ‘template model’, is most likely to be the kinetochore, and this is supported by the finding of sub-maximal levels of Mad2 staining on both the kinetochores of aligned and non-aligned at 6 h after NEB, when the APC is active [17] . However, both a kinetochore-dependent and kinetochore-independent role to the diffusible potent APC inhibitor, the MCC, has been demonstrated, and Mps1 activity is required for both [39] , [40] , [41] . To test if the inhibition of the APC during exit from MI was due to a signal generated at the kinetochore, we took advantage of the large cytoplasmic volume of oocytes and performed bisections. This procedure allows examination of APC activity in the absence of chromosomes and kinetochores. Oocytes, expressing cyclin B1–GFP and histone2B-Cherry, were matured for 4 h after NEB, and then incubated with 400 nM nocodazole, a dose that recruits high levels of Mad2 to kinetochores and activates the SAC [17] . Oocytes were bisected such that two daughter cells of equal size were produced, distinguished by whether or not they contained chromosomes ( Fig. 4a ). In daughter cells possessing the bivalents, the continued presence of nocodazole prevented cyclin B1–GFP degradation over the next hour following bisection ( n =16; Fig. 4b,c ). However, in the anuclear daughter cell, following a ~20-min delay, cyclin B1 degradation was initiated and reached a rate of loss of 68% h −1 ( n =20). This is double the rate normally observed in whole oocytes, but similar to the rate observed in the presence of reversine, ZM447439 or flavopiridol. It is concluded therefore that the continued partial inhibition of the APC during MI is likely generated from kinetochores, as is the canonical SAC, and is consistent with the prevailing ‘template model’. However, the use of the term ‘SAC’ no longer seemed appropriate to describe this inhibition because it is not acting strictly as a checkpoint, but only as a delay to anaphase. This is despite many similarities with the established SAC: a dependency on two of the SAC kinases (Mps1 and Aurora), an integral component of the SAC (Mad2), and the need for the kinetochores. 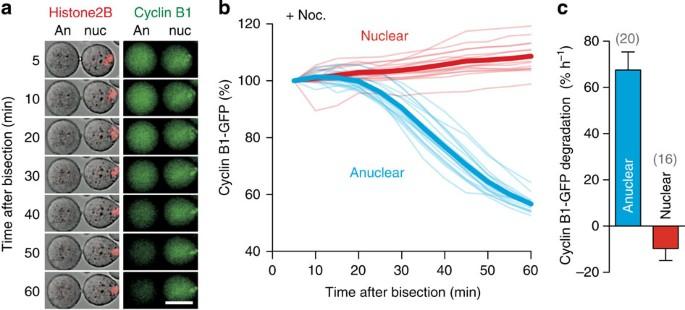Figure 4: Inhibition of the APC by SAC proteins is bivalent dependent. (a) Histone2B-mCherry and cyclin B1–GFP images in two daughter cells following bisection and in the presence of nocodazole. Anuclear halves (an; n=20) degraded Cyclin B1-GFP, while cyclin B1 in nuclear halves (nuc;distinguished by H2B-mCherry labelled bivalents;n=16), was stable. Scale bar, 50 μm. (b) Cyclin B1–GFP levels, normalized at the initiation of imaging after bisection, in nuclear (red) and anuclear (blue) daughter cells. Mean traces are in bold, with individual traces in pale colours. (c) Cyclin B1–GFP degradation rates (mean, s.d.) between 25 and 45 min following bisection. Figure 4: Inhibition of the APC by SAC proteins is bivalent dependent. ( a ) Histone2B-mCherry and cyclin B1–GFP images in two daughter cells following bisection and in the presence of nocodazole. Anuclear halves ( an; n=20 ) degraded Cyclin B1-GFP, while cyclin B1 in nuclear halves ( nuc; distinguished by H2B-mCherry labelled bivalents; n =16), was stable. Scale bar, 50 μm. ( b ) Cyclin B1–GFP levels, normalized at the initiation of imaging after bisection, in nuclear (red) and anuclear (blue) daughter cells. Mean traces are in bold, with individual traces in pale colours. ( c ) Cyclin B1–GFP degradation rates (mean, s.d.) between 25 and 45 min following bisection. Full size image Non-canonical APC inhibition by SAC proteins prolongs MI We decided to investigate what effects there would be on oocytes if the influence of the SAC proteins on the APC were removed during MI exit. If the canonical SAC, operating in prometaphase, was the only time SAC proteins influenced the APC, MI duration would be reduced and this was modelled using cyclin B1–GFP degradation data. The empirical cyclin B1 profile was fitted with a cubic equation ( n =48; R 2 =0.999; Fig. 5a ), whose first differential was plotted to show the rate of change in cyclin B1 degradation with respect to time ( Fig. 5b , green). In order to estimate the length of MI if the APC was maximally active, it was assumed that the oocyte still has to degrade the same total amount of cyclin B1 in order to reduce CDK1 levels sufficiently to permit anaphase. The timing of the onset of APC activity, based on when cyclin B1 degradation is first observed (3.87 h after NEB), was also retained. Therefore, the polynomial was transformed such that its minimum and maximum y values were unchanged, that is, an equal amount of cyclin B1 is degraded, and the value of x i at y =0 on the first differential was preserved because the APC is still switched on at the same time. However, the maximal rate of net cyclin B1 destruction was adjusted to 59% h −1 , a value derived empirically as the rate of cyclin B1 loss following SAC inhibition ( Fig. 2e ). Using this model ( Fig. 5a , red line), the length of MI shortens to 5.8 h if APC activity is not inhibited by SAC proteins during the period of cyclin B1 degradation. Therefore, it is calculated that MI is 2 h longer as a consequence of the persistent influence of SAC proteins (7.8 versus 5.8 h). 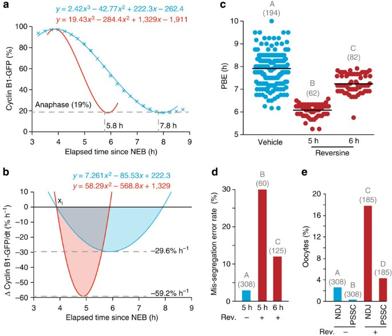Figure 5: Partial and persistent APC inhibition lengthens MI and reduces aneuploidy in metaphase II eggs. (a) Empirical cyclin B1–GFP degradation rates (blue crosses) at the times indicated, used to generate a cubic equation that fits the degradation profile (blue line). Cyclin B1–GFP degradation profile modelled on APC activity that is not inhibited by the SAC during exit from MI (red line). Dashed horizontal line indicates cyclin B1–GFP threshold for anaphase onset, and vertical lines the corresponding timing of anaphase. (b) The rate of change in Cyclin B1-GFP degradation with respect to time during MI. A first differential plot of empirical and modelled cubic equations for the rate of Cyclin B1-GFP degradation. Negative values imply net degradation; horizontal dashed lines, maximal degradation rates;xi, onset of net destruction (first instance ofy=0). (c) Timing of polar body extrusion in oocytes treated with either a vehicle control or reversine at 5 or 6 h after NEB. Black lines indicate means. (d) Chromosome mis-segregation rates in resulting metaphase II eggs following either vehicle or reversine treatment at 5 or 6 h after NEB. (e) NDJ or PSSC rates in resulting eggs following vehicle or reversine addition during MI. (c–e) Numbers of oocytes are indicated in parenthesis; different letters indicate significant difference between groups (P<0.001);c, analysis of variance;d,e, Fisher’s exact test. Figure 5: Partial and persistent APC inhibition lengthens MI and reduces aneuploidy in metaphase II eggs. ( a ) Empirical cyclin B1–GFP degradation rates (blue crosses) at the times indicated, used to generate a cubic equation that fits the degradation profile (blue line). Cyclin B1–GFP degradation profile modelled on APC activity that is not inhibited by the SAC during exit from MI (red line). Dashed horizontal line indicates cyclin B1–GFP threshold for anaphase onset, and vertical lines the corresponding timing of anaphase. ( b ) The rate of change in Cyclin B1-GFP degradation with respect to time during MI. A first differential plot of empirical and modelled cubic equations for the rate of Cyclin B1-GFP degradation. Negative values imply net degradation; horizontal dashed lines, maximal degradation rates; x i , onset of net destruction (first instance of y =0). ( c ) Timing of polar body extrusion in oocytes treated with either a vehicle control or reversine at 5 or 6 h after NEB. Black lines indicate means. ( d ) Chromosome mis-segregation rates in resulting metaphase II eggs following either vehicle or reversine treatment at 5 or 6 h after NEB. ( e ) NDJ or PSSC rates in resulting eggs following vehicle or reversine addition during MI. ( c – e ) Numbers of oocytes are indicated in parenthesis; different letters indicate significant difference between groups ( P <0.001); c , analysis of variance; d , e , Fisher’s exact test. Full size image Increasing APC activity by SAC inhibition raises aneuploidy Does the continued influence of SAC proteins, maintained in MI and associated with measureable lowering of APC activity, have any beneficial function? It is already established that complete loss of the SAC throughout MI in oocytes brings forward the timing of APC activation (equivalent to x i on Fig. 5b ), and this leads to increased chromosome mis-segregation [10] , [12] , [14] , [27] . However, here we have the unusual opportunity to test what appears to be a paradoxical situation, in which we do not interfere with the canonical SAC during prometaphase when it is normally regarded as active, but instead inhibit SAC proteins later when the APC is physiologically most active. Does interfering with SAC proteins only for this period also raise aneuploidy rates? We observed that maturing oocytes treated with the Mps1 inhibitor reversine at either 5 or 6 h after NEB had a shortened progression through MI: by 1.8 h for addition at 5 h after NEB or by 0.7 h when added 1 h later ( P <0.0001, Tukey’s multiple comparison; Fig. 5c ). This acceleration would be expected, because we have now established that MI is being extended by the persistent influence of SAC proteins on the APC. Fully mature metaphase II eggs resulting from these experiments were then in situ spread for aneuploidy analysis. Chromosomally normal mouse eggs contain 20 dyads (a.k.a. sister chromatid pairs). The two major types of segregation error that can be observed in eggs are (i) single chromatids, which are generated by a premature separation of the sister chromatids (PSSC), and (ii) a dyad count that is not 20, which is generated by the homologous chromosome pair co-segregating in MI, this is nondisjunction (NDJ) [42] . Control oocytes, treated with vehicle at either 5 or 6 h after NEB, contained a very low incidence of segregation errors, so the data from the two groups were pooled. The pooled incidence of mis-segregation was 2.6% ( n =308; Fig. 5d ), with a much greater incidence of NDJ over PSSC ( Fig. 5e ). Reversine addition significantly raised chromosome mis-segregation rates to 30.0% ( n =60; P <0.0001, Fisher’s exact test) when added at 5 h after NEB and 12.0% ( n =125; P =0.0002, Fisher’s exact test) at 6 h after NEB; again with far greater numbers of NDJ than PSSC. We assume that higher rates of NDJ are observed following a shortening of MI because the loss or gain of whole bivalents is due to the co-segregation of the non-aligned bivalents previously imaged in live oocytes ( Fig. 1b ). In all cases here, NDJ did result in the separation of the homologue pair, confirming that cohesion cleavage is in itself not dependent on biorientation [43] . The present findings show that the rate of APC-mediated cyclin B1 degradation can be increased two-fold in oocytes when SAC proteins are chemically or immunologically inhibited, or when there are no kinetochores present on which to generate the SAC signal. Such changes in cyclin B1 degradation rate were induced at a time when the APC was normally observed to be maximally active. Therefore, meiotic SAC proteins can be viewed as providing a 50% braking force on APC activity that extends beyond its well-established prometaphase function, where it fully inhibits the APC by generating the so-called ‘wait anaphase’ signal through the MCC. The ability of SAC proteins to reduce APC activity during MI exit ultimately extends its length by 2 h, and importantly this reduces the rate of aneuploidy. Is it possible to estimate the extent to which aneuploidy rates are reduced in oocytes by the influence of SAC proteins on the APC? We have calculated that MI is shortened by 2 h as a result of this influence, with anaphase at ~6 h after NEB. The addition of reversine at 5 h resulted in the same timing of anaphase and raised aneuploidy rates to 30%, but this may be an overestimate given reversine also inhibits erroneous microtubule error correction. In contrast, reversine at 6 h, which would obviously leave error correction during the first 6 h unaffected, leads to 12% aneuploidy rates. This may underestimate the effects of partial inhibition because it does not result in the same profile of cyclin B1 degradation as anticipated by the modelled data, a fact that would impact on the CDK1 profile and so error correction [31] . It is likely therefore that raised APC rates during exit from MI, due to loss of inhibitory SAC protein influence, would raise aneuploidy rates between 12 and 30%. We think it is most likely that the delay to anaphase reduces aneuploidy by allowing more time for erroneous microtubule–kinetochore attachments to be repaired. Such error correction appears especially relevant in oocytes, because bivalents undergo on average three error corrections before establishing biorientation [44] . Importantly, for some bivalents, error correction is still taking place during the final 2 h of MI (here and Lane et al. [17] ). Although much shorter in duration, correction of microtubule–kinetochore attachment also occurs in mitosis during metaphase [45] , [46] . Indeed, it has been suggested that cells may have adapted the length of their metaphase to allow sufficient time for a high proportion of error correction to have taken place before anaphase onset [47] . We speculate that the extensive meiotic error-correcting process explains the continued presence of low levels of SAC proteins on kinetochores during MI [17] , and that this is the basis for the APC inhibition observed here. A previous example, in mitosis, of APC activity in the presence of an active SAC is during ‘mitotic slippage’, an artificially imposed process, where M-phase cells are incubated for prolonged periods by spindle poisons [48] . Recent work has suggested that during such an arrest, the SAC response can be graded, proportional to the amount of Mad2 recruited to kinetochores [8] . Such a finding would be in agreement with the present data in oocytes, where low levels of Mad2 appear to associate with bivalents for the whole period of MI [17] , although the underlying meiotic ‘defect’ on kinetochores allowing such association to remain, needs further investigation. Animals and oocyte culture Four- to six-week-old F1 hybrid mice were obtained from matings of C57Bl6 females with CBA males. These were used for all studies except those involving Fzr1 knockout (Fzr1 −/− ). Fzr1 −/− mice were generated by mating Fzr1 loxp/loxp female mice [49] with Zp3Cre [C57BL/6-Tg(Zp3-cre) 93Knw] males (Jackson Laboratories); and male F1 offspring of the genotype Fzr1 +/loxp /Zp3Cre were mated with Fzr1 loxp/loxp females, to obtain the experiment cohort [50] . All mice were used in accordance with the Australian Code of Practice for the Care and Use of Animals for Scientific Purposes, and were approved by the University of Newcastle Animal Care and Ethics Committee. Oocytes were collected from mice injected with 10 IU equine serum gonadotropin (Invitrogen, New Zealand) in M2 media [51] . Milrinone (1 μM) was added to maintain GV stage arrest [52] . For maturation studies, oocytes were synchronized by incubation in milrinone for 2 h followed by its rapid washout. cRNA manufacture cRNA was transcribed in vitro from purified, linear dsDNA template using a mMessage T3 (H2B-mCherry, cyclin B1–GFP) RNA polymerase kit (Ambion) or T7 (CenpC-GFP) RNA polymerase kit (Promega) [53] . cRNA was suspended in nuclease-free water and its concentration determined by photospectrometry. Microinjection epifluorescence imaging and drug additions cRNA microinjections were conducted in M2 media on the stage of an inverted TE300 microscope (Nikon, Japan), using a 37 °C heated chamber and micromanipulators (Narishige, Japan). cRNA was injected using timed pressure injections from a Picopump (World Precision Instruments) to achieve a size of ~0.2% of oocyte volume, with pipette tip RNA concentrations of 600 ng μl −1 (refs 54 , 55 ). Injection of Mad2 antibody (gift of RH Chen, Taipai) was performed without a holding pipette, instead oocytes were held in place by glass rods present throughout the experiment so as to allow for rapid injection without movement of the oocyte. Antibody was prepared in Hepes-buffered KCl solution, and heat-denatured antibody was heated to 95 °C for 5 min before loading into the injection pipette. Images were captured by epifluorescence using a × 20 objective and CCD camera (Hamamatsu, Japan). Shutters and acquisitions were controlled by micromanager software ( http://www.micro-manager.org ). Drugs were added to media as 10% of the total media volume (100 μl added to 900 μl) to allow rapid mixing. Additions were made immediately following image acquisitions. Final concentrations used were as follows: Reversine (0.1 μM; Sigma), Flavopiridol (5 μM; Sigma), ZM447439 (10 μM; Tocris, USA), Nocodazole (0.4 μM; Sigma). Stock solutions were used at a working dilution of 0.1%. Confocal imaging and chromosome tracking Oocytes injected with Histone 2B-mCherry and CenpC-EGFP cRNA were washed free of milrinone and placed on the stage of an FV1000 confocal microscope equipped with environmental chamber at 37 °C in M2 media covered by mineral oil. Three-dimensional images (17 320 × 320 pixel z-sections with 2-μm spacing; ~34 × 34 × 34 μm) were acquired every 90–300 s using a × 40 objective and × 6 zoom. Images were processed by in-lab ImageJ ( http://www.rsb.info.nih.gov/ij/ ) scripts to determine the centre of mass of the chromosomes and commands returned to the confocal to update subsequent image acquisition such that chromosomes remained in the centre of the field of view throughout maturation. Image processing Images from chromosome tracking experiments ( Fig. 1 ) were generated using ImageJ macros by subtraction of a 2 pixel Gaussian blur from a 10 pixel Gaussian blur background as described elsewhere [44] . Oocyte bisection Oocytes were prepared by removal of the zona pellucida using a brief incubation in acid Tyrode’s solution. Bisections were performed on agar gels made with phosphate-buffered saline and then equilibrated with M2 media under mineral oil. The M2 media contained 0.4 μM nocodazole and 1 mg ml −1 cytochalasin D. Bisection was performed manually under a stereomicroscope using a fine glass fibre. Aneuploidy analysis Matured eggs were treated with monastrol (500 μM; Sigma) to spread chromosomes [56] , [57] before fixation and permeabilization in 1% formaldehyde solution and 0.1% Triton X-100. Fixed eggs were then labelled with CREST serum (1:400; Cortex Biochem, USA) and Hoechst (Sigma) to label kinetochores and chromatin, respectively. Mounted eggs were imaged using a × 60 objective and 0.5 μm z-separation on an FV1000 confocal microscope. Images from different treatment groups were renamed with a numerical code and mixed using in-lab ImageJ software such that chromosome counting was unbiased. Following counting, the software unmixed the images to reveal the aneuploidy rates in different groups. APC activity modelling Empirical cyclin B1 degradation data were entered into Matlab (R2013a, MathWorks, USA) to perform curve fitting. The fitted curve was then adjusted stepwise using a custom-made algorithm until the required maximal APC activity was reached, while the maximal and minimal cyclin B1 levels, and the time of degradation onset, were maintained. Data analysis Fluorescence intensities were recorded from regions of interest encompassing the whole oocytes using ImageJ software and subsequently analysed in Microsoft Excel. Oocytes that did not undergo GV breakdown within 20 min of the modal time, or oocytes with outlying maximal fluorescence intensities were excluded from further analysis. Fluorescence traces were background subtracted and then normalized with maxima at 100%. In experiments where kinase inhibitors or Mad2 antibody were added the individual traces were transformed linearly in the y -axis such that at the time of addition, all traces were equal to 50% fluorescence at the time of intervention. Statistical analysis Statistical analysis was performed using Prism software (GraphPad Software, USA). Analysis of variance was used with Tukey’s multiple comparison test. How to cite this article: Lane, S. I .R. and Jones, K. T. Non-canonical function of spindle assembly checkpoint proteins after APC activation reduces aneuploidy in mouse oocytes. Nat. Commun. 5:3444 doi: 10.1038/ncomms4444 (2014).